Active accumulation of very diluted biomolecules by nano-dispensing for easy detection below the femtomolar range Highly sensitive detection of biomolecules is of paramount interest in many fields including biomedicine, safety and eco-pollution. Conventional analyses use well-established techniques with detection limits ~1 pM. Here we propose a pyro-concentrator able to accumulate biomolecules directly onto a conventional binding surface. The operation principle is relatively simple but very effective. Tiny droplets are drawn pyro-electro-dynamically and released onto a specific site, thus increasing the sensitivity. The reliability of the technique is demonstrated in case of labelled oligonucleotides diluted serially. The results show the possibility to detect very diluted oligonucleotides, down to a few hundreds of attomoles. Excellent results are shown also in case of a sample of clinical interest, the gliadin, where a 60-fold improved detection limit is reached, compared with standard ELISA. This method could open the way to a mass-based technology for sensing molecules at very low concentrations, in environmental as well as in diagnostics applications. The ability to detect biomolecules in highly diluted solutions is of paramount importance in a wide variety of fields, including biomedicine, forensic analysis and environmental monitoring [1] . Nowadays, the immunoaffinitiy-based assays are the methods of choice owing to the high sensitivity and specificity of the antibody–antigen interaction [2] , [3] , [4] . These include well-established techniques such as lateral flow assays (routinely used for urine analysis), and enzyme-linked immunosorbent assays (ELISAs) [5] . They provide relatively quick analysis (that is, few minutes and ~1 h, respectively), however their detection limit (~1 pM) is critical for many frontier applications [6] . Achieving optimal performance for both metrics, rapid analysis and high sensitivity, is still a challenge for any new biosensor. Recently, the detection sensitivity of the immunoassays has been improved by using mainly nanotechnological platforms that make use of surface plasmon resonance [7] , [8] , [9] , surface-enhanced Raman spectroscopy (where surface plasmon resonance enables enhanced Raman scattering) [10] , surface-enhanced Raman spectroscopy combined with superhydrophobic structures [11] , cantilevers [6] , [12] , optical microcavities [13] , nano-mechanical resonators [14] , [15] , nanowires [16] , [17] and integrated microfluidic systems, where typically ion-depletion effects are applied to relatively large volumes of solution [18] , [19] , [20] , [21] . Other particularly attractive techniques are those based on aggregating nanoparticles because they can be easily synthesized in bulk, using standard chemistry techniques, and do not require advanced fabrication approaches (that is, production is bottom-up instead of being top-down). Early work in this field demonstrated colorimetric detection of oligonucleotides using Au nanoparticles functionalized with probe oligonucleotides [22] . Recently, many advances have been reported in this field using different approaches [23] , [24] , [25] , [26] , [27] , [28] , [29] . All of these techniques provide impressive detection sensitivities, down to ~1 fM, but some limitations still exist. First of all, most of these techniques make use of sophisticated and expensive nanotechnology procedures for fabricating and/or manipulating the structures used for binding the analytes [7] , [8] , [9] , [10] , [11] , [12] , [13] , [14] , [15] . Another major drawback, especially in case of the plasmon- and nanoparticle-based approaches, is the diffusion limit and the evaporation-related passive mechanism [10] . Moreover, the surface design is very critical to have the precipitation region of the solute in correspondence of the sensitive area [11] . On the other hand, the microfluidic-based approaches usually employ relatively large volumes of solution (for example, tens of nanolitres) that can be detrimental in several applications. Last, but not least, is the time scale of the analysis that, when operating at low concentrations, is mainly around half an hour or more [6] , [11] . Very recently, alternative techniques have been proposed for concentrating analytes, but still using the passive effects of the evaporation behaviour of sessile droplets [30] , [31] , [32] . Here we show a nano-dispenser (pyro-concentrator, PC) able to draw biomolecules from a mother drop and to accumulate them directly onto the surface of a conventional binding substrate. The technique makes use of a pyroelectric crystal (for example, lithium tantalate) that, while subjected to a thermal gradient, exhibits spontaneous surface charges. The mother drop is exposed to the resulting electric field and, by a well-known electro-hydrodynamic (EHD) effect [33] , is deformed into a Taylor cone from which top tiny droplets (down to tenths of pl) are ejected. This technique has been presented in a previous paper for nozzle- and electrode-free ink-jet printing [34] . Here we demonstrate the possibility of using these tiny droplets for accumulating biomolecules contained in very diluted solutions, pushing the limits of detection down to hundreds of aM. The accumulation effect is achieved directly onto the sample solution by an active mechanism that is free from the time scales of the evaporation effects (as in case of plasmon-based techniques), thus providing a rapid detectability. The nozzle-free modality offers the great advantages of avoiding the dead volume and the clogging issues. Moreover the load volume is in the tenths of microlitre range, contrary to conventional techniques where larger volumes are required (for example, ELISA typically needs 100 μl). Experimental setup The overall experimental setup is depicted schematically in Fig. 1 . 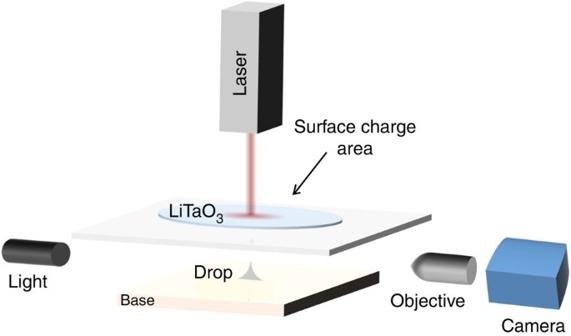Figure 1: Schematic view of the pyro-concentrator. A conventional optical path was used for side visualization of the dispensing process. The scheme is not to scale. Figure 1: Schematic view of the pyro-concentrator. A conventional optical path was used for side visualization of the dispensing process. The scheme is not to scale. Full size image The drop containing the analyte (typically 0.2 μl) is accommodated onto a hydrophobic support. The receiving slide (used for binding the sample molecules) is mounted onto a conventional tilting clamp that ensures the parallel alignment of the two slides, and is equipped with a three-axes translation stage for multiple-site dispensing. A pyroelectric crystal ( z -cut LiTaO 3 and 500 μm thick, UAB Altechna, Vilnius, Lithuania) is mounted onto a separate three-axes translation stage over the receiving slide and drives the EHD-dispensing effect when stimulated by the output beam of a CO 2 laser (wavelength 10.6 μm and output power of 10 W). The CO 2 laser output was modulated by a conventional 5 V transistor-transistor logic (TTL) signal and was equipped with a collinear He-Ne laser beam for precise alignment. According to the pyroelectric effect, an electric field is generated across the thermal-stimulated region of the crystal, thus inducing the pyro-EHD-dispensing effect as described previsously [34] , [35] . A high-speed CMOS camera (Motion Pro Y3-S1; 10,000 frame per s; pixel size 10.85 × 10.85 μm) was used for capturing the dispensing events. The thermal stimulation is impulsive and the pyroelectric crystal reaches temperatures up to about 60 °C, without affecting the molecules, since the pyroelectric crystal is not in contact and safely far from the target substrate. The Supplementary Movie 1 shows a typical liquid bridge occurring in the early stages of operation of the PC, while the Supplementary Movie 2 shows the typical finer bridges and tiny droplets released successively, in conjunction with the decrease of the base volume. The upper part of the images is due to reflection. The movies are shown in slow motion for better visualization. The droplets have volumes that range typically between ~400 pl and ~0.3 pl. The volume was estimated by considering the droplet as a spherical cap. The capability of dispensing very fine droplets is used here for concentrating the molecules dispersed into the sample solution directly onto a limited area of the binding slide by transferring a mother drop of the solution (for example, 0.2 μl) through a series of very small droplets onto the same site. By using labelled molecules it is possible to increase the density of the fluorescence signal and, ultimately, to enhance the sensitivity significantly. The principle of operation is depicted schematically in Fig. 2 . 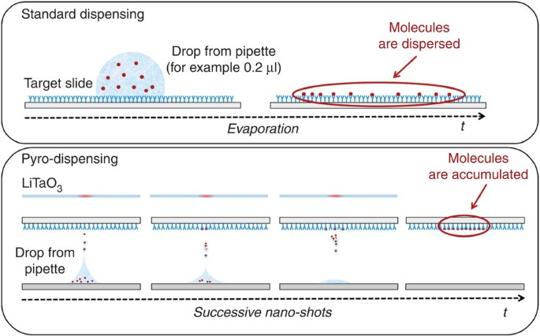Figure 2: Schematic view of the concentration effect. The red dots represent the analyte molecules, the light blue is the buffer and the pendants on the target slide represent the binding species. The scheme is not to scale. Figure 2: Schematic view of the concentration effect. The red dots represent the analyte molecules, the light blue is the buffer and the pendants on the target slide represent the binding species. The scheme is not to scale. Full size image Depositing a specific volume (for example, 0.2 μl) of the solution under test directly onto a binding slide by conventional pipetting, a typical spreading of the drop, followed by buffer evaporation, is expected according to the surface interaction between the liquid and the slide. The solute distributes typically over the contact area of the drop. Conversely, by splitting the mother drop into a series of tiny droplets, and depositing all of them onto a restricted area of the binding slide, the molecules result to be spatially confined over a smaller region, thus augmenting the density of the signal. The process is very quick due to the very fast evaporation of the small-volume droplets. In the framework of commercially available spotter machines, the typical dispensing volumes are in the nl range [36] . Recently, non-conventional technologies have been developed for dispensing smaller droplets, even of biological solutions [37] , [38] . However, the performance of those techniques depends markedly on the application of an external voltage and on the use of a nozzle with consequent detrimental issues related to cross-contaminations, clogging and large dead volumes. One can imagine of dispensing a large number of droplets by a conventional technique (for example, commercial spotter) onto a confined area of the target slide, but the use of pins, nozzles and large dead volumes would require the use of large volumes that in frontier applications are not available (for example, diagnostics of early-stage diseases where only little volumes of sample with very few biomarkers are available). Moreover, the use of nozzles can cause the dispersion of the analyte molecules onto the walls of nozzle and fluidic connections. Here, instead, we demonstrate for the first time the possibility of active accumulation of biomolecules of very dilute solutions directly onto the binding slide through a smart dispensing technique that is free from both electrodes and nozzles. Concentration of oligonucleotides and proteins To demonstrate the performance of the PC, commercially available microarray slides (Supernylon (SN) from Arrayit Corporation, USA) were utilized. The binding capacity of the SN for DNA and proteins is 5 μg per square millimetre and 2 μg per square millimetre, respectively. The molecules to spot were fluorescence labelled and a conventional scanner was used for measuring the fluorescence signal (see Methods). It is worthwhile to mention that in future biosensor application of PC, the slides can be functionalized by specific oligonucleotides or antibodies, thus avoiding pre-labelling of the molecules, and revelation will take place directly on the slide, such as, for example, sandwich ELISA. The fluorescence signal was measured as a function of serial dilutions of an oligonucleotide, labelled in 5′ by Cy5, in case of standard pipetting (single drop of 0.2 μl) and in case of the PC spotting a series of tiny droplets from 0.2 μl mother drop (see Fig. 3 ). These tiny droplets were drawn from the base drop by applying a series of square pulses (150 ms long @ 1 Hz) to the CO 2 laser head. The dilutions of the oligonucleotide solution ranged from 300 nM down to 300 aM. 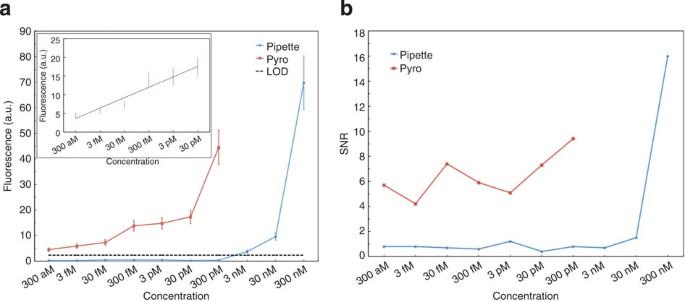Figure 3: Quantitative evaluation of the oligonucleotide spots. Plot of (a) mean fluorescence and (b) SNR as a function of the concentration of spotted oligonucleotides by pipette and by the PC. Each datum inais the mean of 10 replicates and the error bars represent the s.d. from the averages. A total volume of 0.2 μl was dispensed in both cases, but the pipette in one single drop while the PC by a series of tiny droplets. The inset inapresents the linearity range of the PC spots. Figure 3: Quantitative evaluation of the oligonucleotide spots. Plot of ( a ) mean fluorescence and ( b ) SNR as a function of the concentration of spotted oligonucleotides by pipette and by the PC. Each datum in a is the mean of 10 replicates and the error bars represent the s.d. from the averages. A total volume of 0.2 μl was dispensed in both cases, but the pipette in one single drop while the PC by a series of tiny droplets. The inset in a presents the linearity range of the PC spots. Full size image The pipette signal decreases markedly with increasing dilutions and exhibits values of signal-to-noise ratio (SNR) down to around 1 for concentrations below the nanomolar range, and therefore the analyte was undetectable below this concentration. The limit of detection (LOD) was calculated as three times the s.d. of the background intensity. Conversely, the fluorescence signal from the PC shows that ultrasensitive detection is achieved, with SNR values >4, even at concentrations down to hundreds of attomoles, with a linear range from 30 pM to 300 aM ( R 2 =0.9) (see inset in Fig. 3a ). The first concentration utilized by the PC was over the linearity curve probably due to laser scanner settings that were put constant for all of the determinations. The results show that the fluorescence signal of the PC at 300 aM is comparable to that of the pipette spot at 3 nM in terms of signal intensity. In other words, the molecules contained in 0.2 μl of the 300-aM sample (around 36 molecules) were accumulated by the PC into an area of about 0.04 mm 2 and provided a signal equivalent to that of the molecules contained in 0.2 μl of the 3-nM sample (around 4 × 10 8 molecules) dispensed by the pipette over an area about 40 times larger (see Fig. 4a ). 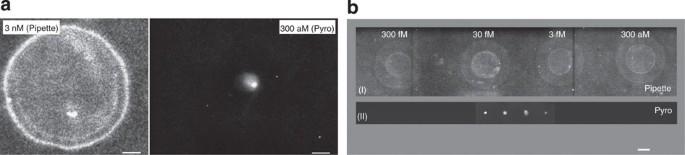Figure 4: Scanner view of the spots. (a) Typical scanner section of a pipette spot at 3 nM (left) and of a PC spot at 300 aM (right), scale bar, 200 μm. (b) Typical scanner sections containing the images of four spots corresponding to most challenging dilutions (from left to right: 300 fM, 30 fM, 3 fM, 300 aM) in case of (I) pipette and (II) PC, scale bar, 800 μm. Figure 4b shows a small section of the scanner images acquired in case of four challenging concentrations of the Cy5 oligonucleotides, for both pipette and PC. Figure 4: Scanner view of the spots. ( a ) Typical scanner section of a pipette spot at 3 nM (left) and of a PC spot at 300 aM (right), scale bar, 200 μm. ( b ) Typical scanner sections containing the images of four spots corresponding to most challenging dilutions (from left to right: 300 fM, 30 fM, 3 fM, 300 aM) in case of (I) pipette and (II) PC, scale bar, 800 μm. Full size image The concentration effect is clearly visible with a significant increment of the fluorescence signal and with about 95% shrinking of the spot area from the pipette to the PC spot. 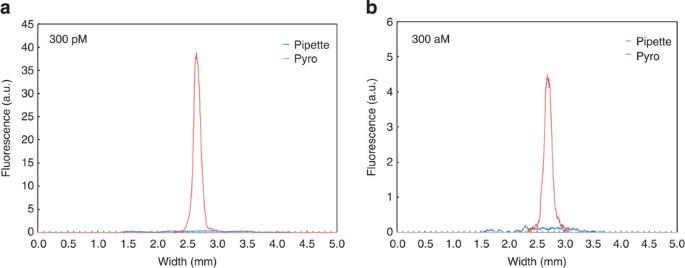Figure 5: Fluorescence profiles of the spots. Typical mean profile of the fluorescence signal of the pipette and of the PC spot in case of (a) 300 pM and (b) 300 aM. Figure 5 shows the fluorescence profiles of the spotted oligonucleotides in case of two edge concentration values (300 pM; 300 aM) and for both methods. The profiles were averaged over the spot area. Figure 5: Fluorescence profiles of the spots. Typical mean profile of the fluorescence signal of the pipette and of the PC spot in case of ( a ) 300 pM and ( b ) 300 aM. Full size image The profiles show clearly that the PC provides a fluorescence signal >100 times larger than the traditional pipette in case of 300 pM and ~40 times larger in case of 300 aM, thus enhancing significantly the detection capability. The PC performance was tested also in case of a protein of clinical interest, the gliadin (see Methods). It is well known that patients with coeliac disease are advised to take a strict gluten-free diet. In the European Union, a maximum level of 20 p.p.m. is allowed for a product declared as ‘gluten free’. Therefore a reliable and high-sensitive technique for assessing the gluten content of food would be of great benefit to patients, dietitians and food manufacturers. The gliadins are the main protein component of the gluten and nowadays they are detected usually by conventional ELISA assays with a LOD ~0.3 p.p.m. (about 30 ng of total protein for 100 μl sample) and a quantification limit (colorimetric test) of about 2 p.p.m. The PC was applied to a range of challenging dilutions of gliadin labelled by Alexa Fluor 647 (see Methods). It is well known that the gliadin is composed of different protein fractions with a wide distribution of molecular weights, and therefore an electrophoretic analysis (lab-on-a-chip) of the labelled gliadin was performed, as shown in Fig. 6 . 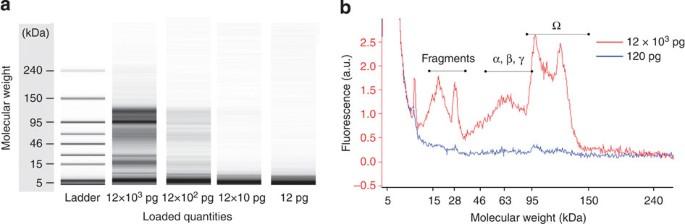Figure 6: Electropherogram of gliadin serial dilutions. (a) Gel-like and (b) fluorescence profile representation. Figure 6: Electropherogram of gliadin serial dilutions. ( a ) Gel-like and ( b ) fluorescence profile representation. Full size image The electropherogram relative to the 12 ng protein per well showed a broad distribution of the molecular weights from 98 to 150 kDa (Ω gliadins), from 46 to 95 kDa (α β γ gliadins) and from 14 to 28 kDa (probably gliadins fragments), which is compatible with a purified preparation of gliadin enriched in Ω gliadins, where no glutenin peaks were observed [39] . It is worth noting that the Ω fraction is mainly responsible for the immune response of coeliac patient and that the fluorescence labelling process depends strictly on the ε amino group of lysine. The gliadins are very poor in lysine content [40] . Therefore the PC data could be influenced negatively by the unfavourable labelling conditions and the performance achieved could be better for protein with high content of lysine. Figure 6 shows the analysis by lab-on-a-chip of 10-fold serial dilutions of labelled gliadin. The signal relative to 120 pg of protein per well resulted to be poorly detectable with respect to the background, thus showing a practical LOD around 1 ng protein per well (250 pg μl −1 sample, 0.25 p.p.m.). Figure. 7a shows the plot of the fluorescence signal obtained in case of the PC as a function of the gliadins dilution factor, while Fig. 7b shows the corresponding fluorescence profiles and scanner images of the PC spots. 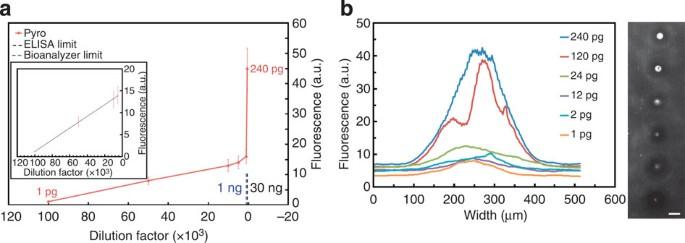Figure 7: Quantitative evaluation of the gliadin spots. (a) Plot of fluorescence of the gliadins spotted by the PC, as a function of the dilution factor and corresponding linearity curve. (b) Mean fluorescence profiles of the PC-spotted gliadins for six dilutions and corresponding scanner image where the dilution grows from top to bottom, scale bar, 300 μm. Each datum inais the mean of 10 replicates and the error bars represent the s.d. from the averages. Figure 7: Quantitative evaluation of the gliadin spots. ( a ) Plot of fluorescence of the gliadins spotted by the PC, as a function of the dilution factor and corresponding linearity curve. ( b ) Mean fluorescence profiles of the PC-spotted gliadins for six dilutions and corresponding scanner image where the dilution grows from top to bottom, scale bar, 300 μm. Each datum in a is the mean of 10 replicates and the error bars represent the s.d. from the averages. Full size image A linear range is clearly visible, as shown in the inset of Fig. 7a ( R 2 =0.8). The results show clearly that the PC is able to detect 1 pg of gliadin (0.2 μl of a solution containing 5 pg μl −1 , 0.005 p.p.m. ), thus reaching 60-fold improvement compared with current limits of ELISA assays (0.3 p.p.m.) and comparable to a very sensitive (0.006 p.p.m.) approach to gliadin determination recently described in literature [30] , thus opening the way to high-sensitive detection. In conclusion, the capability of the PC of dispensing tiny droplets allowed us to overcome the current limits in detecting biomolecules in very diluted solutions, with detection limits down to hundreds of aM. The PC was applied for detecting proteins of clinical interest (gliadins), showing 60-fold improvement compared with the standard LOD of ELISA. The technique breaks through the limitations of drop diffusion that are encountered typically in case of those passive methods that make use of drop evaporation over functionalized substrates (for example, plasmonics), thus opening the way to a variety of revolutionary advantages in the field of biosensors. The detection time scale is reduced significantly and the dead volume issue is totally avoided. The load volume is extremely reduced (200 nl versus 100 μl in ELISA), that is of great importance in all of those applications where the target solution is available only in small quantities. The contact-free procedure avoids cross-contaminations, intermediate washing protocols and time-consuming additional procedures. For example, in case of plasmon-based techniques, a specific functionalization has to be performed for each kind of molecule under investigation, contrary to our system that can accommodate any desired pre-functionalized surface. To summarize, the technique provides a series of advantages compared with other frontier methods proposed in literature: (1) ultra-high sensitivity, (2) active mechanism, (3) rapidity, (4) adaptability to standard detection protocols, (5) reduced reaction volumes, (6) reduced sample preparation complexity, (7) ready reusability, (8) free from functionalization and (9) reduced load volume. We envisage the potential application of this technique for highly sensitive biosensors useful for biomedicine as well as for controlling environmental pollutions or hazards. Test analytes 5′ Cy5 ( λ ex ~650 nm; λ em ~670 nm) fluorescence-labelled oligonucleotide (5'-CGCGATCCCACCCAGGGAGCCACTGAGATGATGGCG-3′, 66.7% G-C content, MW 12,131 g mol −1 ) was synthesized at Eurofins mwg/operon—Ebersberg-D. region. The oligonucleotide was solubilized in Tris-EDTA buffer at initial concentration of 100 μM. A 300-nM stock solution was prepared and serial dilutions in Tris-EDTA were used. The samples were mixed with an advanced buffer system (Micro-Spotting Solution Plus 2X, ArrayIt), in a ratio 1:1, to improve the surface properties of the oligonucleotide samples deposited during printing. The analyte solution (0.2 μl) was deposited onto the base support by a Hamilton Modified Microliter Syringe (7000 Series). The gliadin sample (Sigma) was provided kindly by Dr S. D’Auria, CNR-IBP. One mg of gliadin was solubilized in 1 ml of phosphate-buffered saline and 0.1 M sodium bicarbonate solution was added to raise the pH of the reaction mixture to 8–8.5. A volume of 100 μl of solution was labelled using the Alexa Fluor 647 Antibody Labelling Kit (Molecular Probes, Invitrogen) following the manufacturer’s instructions. The reaction mixture was loaded onto a spin column (available with the kit), containing a gel-filtration resin in phosphate-buffered saline (pH 7.2), and after centrifugation at 1,100 g for 5 min, the labelled protein (~100 μl) was collected in a tube, while the band of unreacted dye was retained in the void volume. The concentration of labelled gliadin (610 ng ml −1 ) was calculated measuring the adsorbance at 280 nm and subtracting the adsorbance at 650 nm correct by a 0.03 factor, to eliminate the contribution of lysine-linked dye. SN slides SN slides were purchased from Arrayit Corporation. They consist of a glass microscope slide (25 × 76 × 1) mm 3 coated with a positively charged nylon membrane, around 150 μm thick. Binding capacity for DNA: 5 μg per square millimetre. Binding capacity for proteins: 2 μg per square millimetre. Reaction area: (25 × 76) mm 2 . The surface is positively charged to allow direct crosslinking of DNA and proteins to the surface. Scanner A conventional fluorescence scanner InnoScan 710 (Innopsys, Carbonne, France) was used for reading the slides. Main scan parameters: laser source at 635 nm and 10 mW power; pixel size 3 μm and scan speed of 10 lines s −1 ; detection gain 25% PMT. These settings guaranteed a photometric performance with a sensitivity of minimum 0.05 fluorescent molecules per μm 2 and an optical resolution of 2.7 μm. The 16-bit images captured by the scanner were evaluated quantitatively by Mapix software V5.5.0 (Innopsys). Lab-on-chip electrophoresis Electrophoresis analysis of gliadin labelled by Alexa Fluor 647 was performed using a 2100 Bioanalyzer equipped with a 2100 Expert Software and the Protein 250 High Sensitivity kit (Agilent Technology, Santa Clara, CA, USA), following the manufacturer’s instructions. The gliadin was diluted to a concentration of 3.05 ng μl −1 (1/200 in distilled water of mater solution) and 3 serial dilutions 1/10 were prepared. Four μl for each sample, combined with 2 μl denaturing solution (non-reducing conditions) were treated at 98 °C for 5 min, cooled down and the complete volume 6 μl was loaded into each sample well. How to cite this article: Grilli, S. et al. Active accumulation of very diluted biomolecules by nano-dispensing for easy detection below the femtomolar range. Nat. Commun. 5:5314 doi: 10.1038/ncomms6314 (2014).